ParaHydrogen Induced Polarization of13C carboxylate resonance in acetate and pyruvate The advent of nuclear spins hyperpolarization techniques represents a breakthrough in the field of medical diagnoses by magnetic resonance imaging. Dynamic nuclear polarization (DNP) is the most widely used method, and hyperpolarized metabolites such as [1- 13 C]-pyruvate are shown to report on status of tumours. Parahydrogen-induced polarization (PHIP) is a chemistry-based technique, easier to handle and much less expensive in respect to DNP, with significantly shorter polarization times. Its main limitation is the availability of unsaturated precursors for the target substrates; for instance, acetate and pyruvate cannot be obtained by direct incorporation of the parahydrogen molecule. Herein we report a method that allows us to achieve hyperpolarization in this kind of molecule by means of a tailored precursor containing a hydrogenable functionality that, after polarization transfer to the target 13 C moiety, is cleaved to obtain the metabolite of interest. The reported procedure can be extended to a number of other biologically relevant substrates. Recent years have witnessed a renewed interest in routes to hyperpolarization as a means of overcoming sensitivity issues associated with magnetic resonance spectroscopy and magnetic resonance imaging (MRI). In this context, most attention has been devoted to the application of the dissolution DNP (dynamic nuclear polarization) methodologies [1] , [2] , [3] . Applications of DNP have led to very important results in the field of metabolic MRI. It has been shown that the administration of hyperpolarized 13 C-labelled substrates such as pyruvate [2] , [3] , lactate [4] , [5] , fumarate [6] , acetate [7] , [8] and bicarbonate [9] , [10] can report on their intracellular transformations, providing outstanding information for early detection of pathologic states and for their response to therapy [11] . A limitation to the widespread use of this approach relies on the fact that it requires access to complex and expensive instrumentation, available only in a limited number of laboratories. Moreover, the DNP methodology requires relatively long times for the polarization step with consequent large consumption of cryogenic liquids. An alternative route to hyperpolarized molecules is represented by parahydrogen-induced polarization (PHIP) [12] , [13] that has the advantage of being cheaper and easier to handle with respect to DNP. As far as biomedical applications are concerned, few molecules have been hyperpolarized by means of this method. Among them, succinate [14] , [15] and phospho-lactate [16] , [17] are the only metabolites for which good hyperpolarization level has been achieved until now. Alternative routes have been proposed to achieve PHIP on biologically relevant molecules by functionalizing the substrates of interest with moieties capable of hydrogenation [18] , [19] , [20] . However, the structural modifications introduced by the unsaturated group may significantly alter their biological behaviour with respect to the native substrates. An attempt to tackle the major limitations of PHIP has been pursued with the recently introduced signal amplification by reversible exchange method [21] , [22] , [23] . With this approach, parahydrogen protons are not added to the substrate but the hyperpolarization transfer takes place on a transient adduct formed by the substrate, parahydrogen and the organometallic complex. This method has been successfully tested on several biologically relevant molecules such as pyrimidines, purines, amino acids and drugs [24] , [25] . However, in vivo application still suffers from low polarization levels and the need for suitable organometallic complex to efficiently renew hyperpolarization [26] . As far as PHIP is concerned, efficient polarization transfer from parahydrogen spin order to 13 C longitudinal magnetization of carbonyl groups can be achieved by the addition of the para-H 2 molecule to a double or a triple bond adjacent to the carbonyl group [23] . The amount of polarization transferred from parahydrogen protons (A and A′) to heteronuclear resonances (X) (that is, 13 C) depends on the coupling asymmetry of the two parahydrogen protons with the X nucleus ( J AX - J A′X /2* J AA′ ) [27] , [28] . Therefore, heteronuclear polarization cannot be achieved if the target X nucleus is symmetrically coupled with the two protons. Moreover, polarization is expected to be low if the difference between J AX and J A′X is small or when the moiety to be hydrogenated is far away from the heteroatom. Optimal polarization transfer has been observed when the added parahydrogen protons are two and three bonds away from the ‘target’ heteronucleus ( Fig. 1 , structure a ). 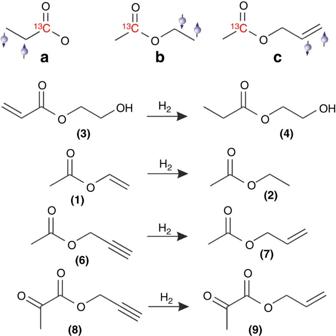Figure 1: Unsaturated substrates and hydrogenation reactions. The molecules considered in this work differ for the number of bonds between the13C-carbonyl moiety and the site of para-H2addition. This is schematically shown in the upper part of the figure fora,bandcstructures. Previously published PHIP work has mainly dealt with typeacompounds. The specific parahydrogenation reactions and the obtained products (with the numbers used in the text) are reported in the lower part of the figure. Figure 1: Unsaturated substrates and hydrogenation reactions. The molecules considered in this work differ for the number of bonds between the 13 C-carbonyl moiety and the site of para-H 2 addition. This is schematically shown in the upper part of the figure for a , b and c structures. Previously published PHIP work has mainly dealt with type a compounds. The specific parahydrogenation reactions and the obtained products (with the numbers used in the text) are reported in the lower part of the figure. Full size image Herein we report PHIP results showing that high polarization levels can also be achieved from the reaction of para-H 2 with substrates having general formula b and c ( Fig. 1 ). Moreover, a successive hydrolysis step yields hyperpolarized carboxylic acids, such as acetate and pyruvate whose formation has been till now precluded by the lack of suitable dehydrogenated precursors. PHIP of acetate The 13 C-NMR spectrum acquired immediately after the parahydrogenation of vinyl acetate ( 1 ) (1.1% C-13), carried out at earth’s magnetic field, according to the ALTADENA method [29] , showed hyperpolarized signals for the aliphatic carbons of ethyl acetate ( 2 ), whereas no polarization was observed at the 13 C carboxylate carbon ( Fig. 2 , the whole spectrum is reported in Supplementary Fig. 1 ). Conversely, the application of low magnetic field cycling [30] , [31] immediately after the parahydrogenation reaction yielded an efficient polarization transfer to the 13 C longitudinal magnetization of the carboxylate group ( Fig. 2 , for the whole spectrum see Supplementary Fig. 2 ). 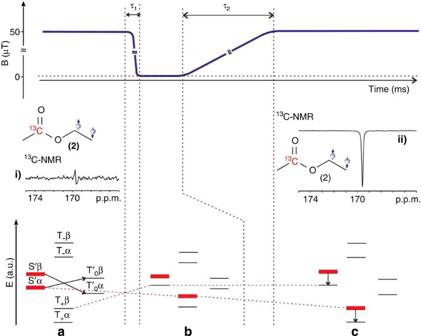Figure 2: Field cycling yield high polarization on13C carboxylate signal of ethyl acetate. Upper part of the figure: magnetic field profile during the field cycle. The magnetic field is cycled between earth magnetic field, where the parahydrogenation reaction is carried out, and nearly zero field by using concentric cylinders made of μ-metal. The first passage from earth to zero field is fast (non-adiabatic) (τ1); the second passage is slow (adiabatic) and takes about 5 s (τ2). Central part of the figure:13C spectrum (one scan, carbonyl region only) of ethyl acetate obtained from parahydrogenation of vinyl acetate (85 mM), acquired at 14.1 T and 298 K, before the application of field cycle (i) and after application of field cycling (ii). Ini, the13C carboxylate signal is hardly detectable from the spectral noise; inii, the same carbonyl resonance shows high polarization. Lower part of the figure: spin states of the AA’X system and their populations immediately after parahydrogen addition (a), after non-adiabatic transport to low field (b) and successive adiabatic transport to earth field (c). The parahydrogenation experiments were repeated three times. Figure 2: Field cycling yield high polarization on 13 C carboxylate signal of ethyl acetate. Upper part of the figure: magnetic field profile during the field cycle. The magnetic field is cycled between earth magnetic field, where the parahydrogenation reaction is carried out, and nearly zero field by using concentric cylinders made of μ-metal. The first passage from earth to zero field is fast (non-adiabatic) ( τ 1 ); the second passage is slow (adiabatic) and takes about 5 s ( τ 2 ). Central part of the figure: 13 C spectrum (one scan, carbonyl region only) of ethyl acetate obtained from parahydrogenation of vinyl acetate (85 mM), acquired at 14.1 T and 298 K, before the application of field cycle ( i ) and after application of field cycling ( ii ). In i , the 13 C carboxylate signal is hardly detectable from the spectral noise; in ii , the same carbonyl resonance shows high polarization. Lower part of the figure: spin states of the AA’X system and their populations immediately after parahydrogen addition ( a ), after non-adiabatic transport to low field ( b ) and successive adiabatic transport to earth field ( c ). The parahydrogenation experiments were repeated three times. Full size image Support for the view that the polarization level attained for the 13 C carboxylate group of ethyl acetate is good was obtained by the parahydrogenation of hydroxyethyl acrylate ( 3 ) to hydroxyethyl propionate ( 4 , HEP). The PHIP effect on the 13 C carboxylate signal of HEP had been previously estimated to yield polarization level as high as 20% [31] . As shown in Fig. 3 , the polarization level observed for the 13 C carboxylate resonances of ethyl acetate ( 2 ) and HEP ( 4 ) are quite similar. 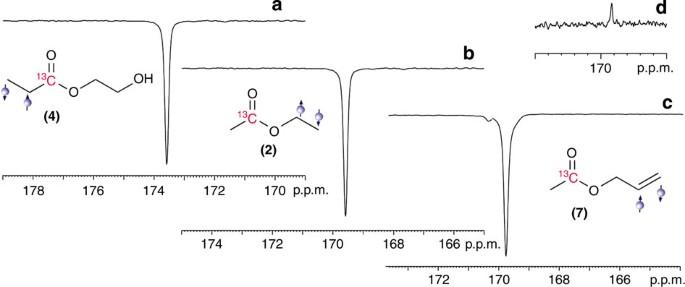Figure 3: C-13 carboxylate hyperpolarization on type A, B and C molecules. Similar level of hyperpolarization is obtained on field cycle application, irrespective of the position where parahydrogens are added, that is (a) at the adjacent position to the carboxylate (hydroxy ethyl propiolate,4), (b) at three–four (ethyl acetate,2), (c) or at four–five (acetic acid allyl ester7) bonds far away from the carboxylate13C atom. (d) Thermal equilibrium spectrum of acetic acid allyl ester, 10,100 scans (30° pulse, 15 h acquisition time). The concentration of the three precursors was the same, that is, 85 mM. The parahydrogenation reaction was carried out in acetone-d6. All the parahydrogenation experiments were repeated three times. Figure 3: C-13 carboxylate hyperpolarization on type A, B and C molecules. Similar level of hyperpolarization is obtained on field cycle application, irrespective of the position where parahydrogens are added, that is ( a ) at the adjacent position to the carboxylate (hydroxy ethyl propiolate, 4 ), ( b ) at three–four (ethyl acetate, 2 ), ( c ) or at four–five (acetic acid allyl ester 7 ) bonds far away from the carboxylate 13 C atom. ( d ) Thermal equilibrium spectrum of acetic acid allyl ester, 10,100 scans (30° pulse, 15 h acquisition time). The concentration of the three precursors was the same, that is, 85 mM. The parahydrogenation reaction was carried out in acetone- d 6 . All the parahydrogenation experiments were repeated three times. Full size image After the polarization transfer step the ethyl group was removed by hydrolysis, while the hyperpolarization is kept on the 13 C carboxylate signal of acetate ( 5 ). Hydrolysis was carried out by adding sodium hydroxide (1 M solution) to the reaction mixture (parahydrogenation in water) and hyperpolarized 13 C acetate ( 5 ) is instantaneously formed ( Fig. 4 ). 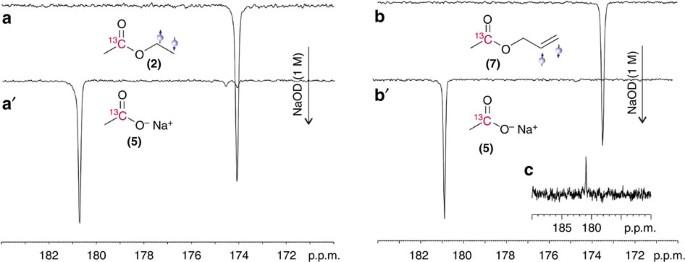Figure 4: Formation of13C-hyperpolarized acetate. Free13C-hyperpolarized acetate (13C natural abundance) is obtained from hydrolysis of parahydrogenated ethyl (2, spectruma) and allyl (7spectrumb) esters (reactions carried out in aqueous medium). Addition of sodium hydroxide (1 M) to the aqueous solutions of ethyl acetate and acetic acid allyl ester allows efficient hydrolysis with the release of the alcoholic moiety, whereas polarization is fully maintained on the carbonyl moiety (a’,b’). (c)13C spectrum of the acetate product at thermal equilibrium, 1,000 scans (90° pulse), acquisition time 56 h. The parahydrogenation experiments were repeated three times. Figure 4: Formation of 13 C-hyperpolarized acetate. Free 13 C-hyperpolarized acetate ( 13 C natural abundance) is obtained from hydrolysis of parahydrogenated ethyl ( 2 , spectrum a ) and allyl ( 7 spectrum b ) esters (reactions carried out in aqueous medium). Addition of sodium hydroxide (1 M) to the aqueous solutions of ethyl acetate and acetic acid allyl ester allows efficient hydrolysis with the release of the alcoholic moiety, whereas polarization is fully maintained on the carbonyl moiety ( a ’, b ’). ( c ) 13 C spectrum of the acetate product at thermal equilibrium, 1,000 scans (90° pulse), acquisition time 56 h. The parahydrogenation experiments were repeated three times. Full size image As the synthesis of the vinyl esters is not straightforward due to keto-enol tautomerism of ethanol and ethanal species, propargylic ester was considered. Acetic acid prop-2-ynyl ester ( 6 ) was synthesized, reacted with para-H 2 and the obtained acetic acid allyl ester ( 7 ) was subjected to the field cycling procedure. The hyperpolarization level obtained on the 13 C carboxylate signal of 7 was similar to that observed for the corresponding vinyl ester. Again, hydrolysis yielded the free acid by maintaining a good polarization level of the parent ester ( Fig. 4 ). When the deuterated propargylic alcohol was used (2-d 2 propargylic alcohol) [19] polarization transfer to 13 C carboxylate signal was not obtained (spectrum in Supplementary Fig. 3 ). PHIP of pyruvate On the basis of the results obtained on propargylic ester of acetate, propargyl alcohol was used to prepare the unsaturated ester of pyruvic acid 2-propynyl-2-oxopropanoate ( 8 ) [32] (naturally abundance [1- 13 C] pyruvate). According to the reported phase transfer procedure [33] , hydrogenation of the ester was carried out in a chloroform (90%)–methanol (10%) mixture and was followed by the addition of an aqueous basic solution (NaOD 1 M). Two phases quickly separated out, the catalyst being retained in the organic phase, while the hyperpolarized sodium salt was extracted in the aqueous phase. This method results in an improved hydrogenation efficiency with respect to hydrogenation in water and yielded an aqueous solution of the polarized metabolite free from the organometallic catalyst. As shown in Fig. 5 , a good level of polarization was observed for the C-13 carboxylate signals of the allyl ester of pyruvate ( 9 ), on the application of the magnetic field cycling (thermal equilibrium 13 C and 1 H NMR spectra of the natural abundance C-13 carbonyl and acetal tautomer are reported in Supplementary Figs 4 and 5 ). 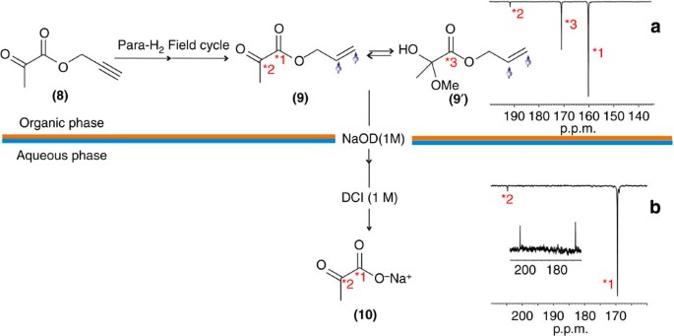Figure 5: Formation of13C-hyperpolarized pyruvate. Organic phase: parahydrogenation of 2-propynyl-2-oxopropanoate (8) carried out in chloroform/methanol (10:1) and field cycling allow hyperpolarization of the13C carboxylate of the allyl ester of pyruvate (a):13C spectrum, one scan). The presence of methanol in the reaction mixture causes an equilibrium between carbonylic (9) and emi-acetalic (9’) forms. All the carbonyl signals (1, 2 and 3) are hyperpolarized. Hydrolysis was carried out by means of the addition of NaOD (1 M), then DCl (1 M solution) was added to reach pH 5. The aqueous phase was collected in a NMR tube, the13C-NMR single scan spectrum (b) showed polarized signals of sodium pyruvate (10) (~50 mM). Thecspectrum is the corresponding thermal equilibrium spectrum acquired with 10,100 scans (30° pulse, Ernst angle, acquisition time 15 h 20′). The parahydrogenation experiments were repeated three times. Figure 5: Formation of 13 C-hyperpolarized pyruvate. Organic phase: parahydrogenation of 2-propynyl-2-oxopropanoate ( 8 ) carried out in chloroform/methanol (10:1) and field cycling allow hyperpolarization of the 13 C carboxylate of the allyl ester of pyruvate ( a ): 13 C spectrum, one scan). The presence of methanol in the reaction mixture causes an equilibrium between carbonylic ( 9 ) and emi-acetalic ( 9 ’) forms. All the carbonyl signals (1, 2 and 3) are hyperpolarized. Hydrolysis was carried out by means of the addition of NaOD (1 M), then DCl (1 M solution) was added to reach pH 5. The aqueous phase was collected in a NMR tube, the 13 C-NMR single scan spectrum ( b ) showed polarized signals of sodium pyruvate ( 10 ) (~50 mM). The c spectrum is the corresponding thermal equilibrium spectrum acquired with 10,100 scans (30° pulse, Ernst angle, acquisition time 15 h 20′). The parahydrogenation experiments were repeated three times. Full size image Next, hydrolysis and phase separation were quickly carried out by adding NaOD (1 M) and the pH of the solution was finally set to about 5 by the addition of an equimolar amount of DCl. Overall, this procedure took about 10 s. The 13 C spectrum of the aqueous phase ( Fig. 5 ) shows that a good polarization level is maintained on pyruvate ( 10 ) after hydrolysis and pH equilibration. The relaxation times (T 1 ) of the 13 C carboxylate signals of allyl pyruvate ( 9 ) and pyruvate ( 10 ) were measured, at 14.1 T, to be T 1 =33.5±5′′ and T 1 =40±6′′, respectively. The occurrence of such a long T 1 s ensured that polarization loss during the experimental work-up is limited. The results reported herein show that PHIP can be obtained on molecules, such as acetate ( 5 ) and pyruvate ( 10 ) (and, in principle, can be extended to other carboxylic acids), by using precursors containing a side arm capable of hydrogenation that can be hydrolysed to yield the hyperpolarized target products. The reported method, named PHIP-SAH (PHIP by means of side arm hydrogenation) relies on the following steps: (i) functionalization of the target acidic molecule with an unsaturated alcoholic group (vinyl/propargyl alcohol); (ii) parahydrogenation of the unsaturated ester; (iii) polarization transfer to the carboxylate C-13 signal by applying magnetic field cycling; (iv) release of the alcohol moiety by hydrolysis to obtain the polarized 13 C-carboxylate-containing product. Parahydrogenation of vinyl acetate ( 1 ) and hydrolysis have been previously reported [34] for obtaining hyperpolarized ethanol. Here it is shown that polarization transfer to the 13 C carboxylate signal is possible by means of magnetic field cycling. It was reported [31] that magnetic field cycling yields about 20% polarization on HEP ( 4 ) and it is shown in this work that the same polarization level is obtained in parahydrogenated ethyl acetate ( 2 ), in spite of less favourable J coupling pattern. Polarization transfer from the two parahydrogen protons (indicated with A and A′) to the 13 C carboxylate signal (X) of ethyl acetate ( 2 ) may be accounted for on the basis of spin state populations. Spin states are expressed as product of ortho ( αα = T + , ( αβ + βα )= T 0 , ββ = T − )-para (( αβ − βα )= S ) states for the protons, and α and β states for 13 C (ref. 27 ). When the parahydrogen molecule is added to the 13 C-containing substrate, at the earth’s magnetic field, the singlet ( S ) and the triplet ( T 0 ) states are mixed, thanks to asymmetric coupling of the protons with the heteroatom. The states S ′ α - T 0 ′ α (for 13 C in the α -state) and S ′ β - T 0 ′ β (for 13 C in the β -state) are formed, where the prime indicates that these states are a linear combination of S and T 0 states with a dominating singlet ( S ′) or triplet ( T 0 ′) character ( Fig. 2 , lower part, a ) [27] . Singlet–triplet mixing allows transitions between levels S ′ α - T 0 ′ β (polarized absorption) and S ′ β - T 0 ′ α (polarized emission), and the transition probability can be calculated from the relevant J coupling values. For ethyl acetate ( 2 ) ( J AX =3.2 Hz, J A′X =1.7 Hz and J AA′ =7.5 Hz) the resulting transition probability is , while for hydroxyl ethyl propiolate ( 4 ) ( J AX =7.2 Hz and J A′X =−5.6 Hz J AA′ =7.5 Hz) the transition probability is 0.37 (detailed calculations are reported in Supplementary Methods ). As polarization intensity is also related to the population difference between levels, which is 0.51 for HEP ( 4 ) and 0.98 for ethyl acetate ( 2 ), it can be derived that polarization on the 13 C carboxylate signal of parahydrogenated ethyl acetate is expected to be only ~10% of that on HEP, in agreement with what was anticipated from the J coupling ratio ( J AX - J A′X /2* J AA′ ). When magnetic field cycling is applied, isotropic mixing between heteronuclei takes place at nearly zero field and all the states with the same total spin T + β - T 0 α - Sα ( I =−1/2) and T − α - T 0 β - Sβ ( I =+1/2) are mixed. Owing to non-adiabatic passage from earth’s field to low field, the most stable state (state T + β at earth’s field) becomes the most populated state ( Fig. 2b and Supplementary Fig. 6 ). If J couplings of ethyl acetate ( 2 ) are considered, almost all the singlet state population is transferred to the state T + β while, on HEP ( 4 ) the singlet state population is shared between the three states ( Supplementary Methods ). Then, when the sample is adiabatically transferred back to high field, the spin state populations are maintained and the hyperpolarized 13 C transitions take place between the states T + β − T + α and S′β – S′α ( Fig. 2c ). Note that, in this case, the transition probability is and polarization intensity is only due to population differences. The intensity of hyperpolarized longitudinal magnetization of the 13 C carboxylate signal of ethyl acetate is expected to be even higher than that for HEP (for more detail, see the Supplementary Information , Methods). Therefore, it may be expected that high polarization levels can be obtained on 13 C carboxylate signals of the esters precursors using a finely controlled field cycling procedure [31] . When propargyl esters are used, polarization transferred to the 13 C-carbonyl signal is the same as that obtained for the vinyl ester, albeit the parahydrogen protons are further from the 13 C carboxyl atom. We surmise that, in this case, parahydrogen spin order is transferred to the methylenic protons and, from these protons, to the 13 C carboxylate atom. The lack of polarization on the 13 C carboxylate signal obtained when the deuterated compound is used supports this hypothesis. In summary, these findings open a very interesting perspective for the use of parahydrogen-based procedures for the generation of hyperpolarized, biologically relevant, molecules. The possibility of using propargyl alcohol as a removable synthon to generate PHIP on 13 C resonances markedly widens the applicability of the PHIP approach. The access to hyperpolarized molecules by means of the easy-to-implement PHIP-SAH procedure is expected to promote renewed interests in the field of magnetic resonance spectroscopy–MRI hyperpolarization that have been precluded by the high cost and complexity of the DNP methodology. Chemicals Vinyl acetate ( 1 ), hydroxyl ethyl propiolate ( 2 ) and the catalyst [Rh(1,4-bis(diphenylphosphino)butane)(cyclooctadiene)][BF 4 ] were purchased from Sigma-Aldrich and used without purification. Propargyl esters of acetic acid and pyruvic acid ( 5 and 7 ) were synthesized as reported in ref. 33 and used without further purification. The water-soluble catalyst [Rh(norbonadiene)1,4-bis-[(phenyl-3-propane sulfonate) phosphine][BF 4 ] (3 mM) was prepared according to the method described by Hövener et al . [35] Parahydrogenation experiments Parahydrogenation of hydroxyethyl acrylate ( 3 ), vinyl acetate ( 1 ) and propargyl acetate ( 6 ) were carried out in acetone- d 6 using the commercial catalyst [Rh(1,4-bis(diphenylphosphino)butane)(cyclooctadiene)][BF 4 ]. NMR tubes (5 mm) equipped with Young valve were charged with the catalyst (4 × 10 −3 mmol), 400 μl of acetone- d 6 , and the catalyst was activated by hydrogenation of the coordinated diene. The substrate was added (35 × 10 −3 mmol) and the tube pressurized with 2 bar of parahydrogen, while keeping it in liquid nitrogen, to achieve a higher parahydrogen pressure in the NMR tube and to freeze the hydrogenation reaction. The NMR tube was then thawed to room temperature and vigorously shaken for about 10′′. Immediately after shaking, the sample was (a) placed in the NMR spectrometer (Bruker Avance 600 MHz 1 H-NMR) and a single scan 13 C spectrum was acquired or, alternatively, (b) quickly dropped in the μ-metal shield, slowly taken out of it (about 5′′) and immediately placed in the NMR spectrometer for 13 C acquisition (one scan). For the parahydrogenation in aqueous medium, 400 μl of the catalyst [Rh(norbonadiene)1,4-bis-[(phenyl-3-propane sulfonate) phosphine][BF 4 ] (3 mM) prepared according to the reported procedure [35] were placed into the 5-mm NMR tube equipped with Young valve, the substrate was added (35 × 10 −3 mmol) and the tube pressurized with 2 bar of parahydrogen, while keeping it in liquid nitrogen. After thawing, the NMR tube was warmed up using a water bath (90 °C) for 5′′. Then, the parahydrogenation reaction was initiated by shaking the tube and field cycle was applied as described for the reaction in organic medium. For phase extraction experiments, 10 mm NMR tubes equipped with Young valve were used. The catalyst [RhCOD(dppb)][BF 4 ] (4 × 10 −3 mmol) was activated in 50 μl of methanol- d 4 , 500 μl of CDCl 3 and the substrate 2-propynyl-2-oxopropanoate (50 × 10 −3 mmol) was added. The NMR tube was pressurized with 2 bar of parahydrogen, while keeping it in liquid nitrogen, then it was thawed and warmed up by means of a water bath (90 °C). Parahydrogenation and field cycle were applied as described above, then the NMR tube was opened and 300 μl of NaOD solution (1 M) were added to the organic solvent, followed few seconds later by the addition of 300 μl of DCl (1 M). The aqueous phase is then transferred into a 5-mm NMR tube and placed into the NMR spectrometer (Bruker Avance 600 MHz) for the acquisition of the 13 C spectrum (one scan). Field cycling Two concentric μ-metal cylinders (200 mm height, 30 and 50 mm diameter) (Meca-Magnetic, Amilly, France) were used to carry out field cycling experiments. NMR tubes were dropped into the centre of the shield and then slowly pulled up out of the cylinders in about 5′′. Parahydrogen Hydrogen gas was enriched to 92% parahydrogen by catalytic conversion at low temperature (36 K) using a Bruker parahydrogen generator (BPHG) and collected directly into the NMR tubes for parahydrogenation reactions. How to cite this article : Reineri, F. et al . ParaHydrogen Induced Polarization of 13 C carboxylate resonance in acetate and pyruvate. Nat. Commun. 6:5858 doi: 10.1038/ncomms6858 (2015).